RETRACTED ARTICLE:The Arabidopsis NOT4A E3 ligase promotes PGR3 expression and regulates chloroplast translation 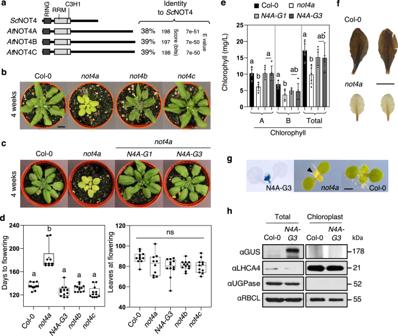Fig. 1: Identification of NOT4-like proteins in Arabidopsis. aSchematic diagram of protein domain structure and % amino acid identity forSachharomyces cerevisiae(Sc) andArabidopsis thaliana(At) NOT4 proteins. For full sequence alignments see Supplementary Fig.1.b,cRepresentative rosette images of 4-week-old col-0,not4a-cmutants, and two independentnot4acomplementation lines (N4A-G1andG3) grown under long day (LD) conditions. Bar = 1 cm.dDays to flowering and rosette leaf number at flowering for genotypes shown under short-day (SD) conditions (n= 10–12 per genotype). Box and whiskers plots show max and min, 25–75th percentiles (box), median (line) and mean (+). Letters indicate one-way ANOVA; Tukey’s test (p< 0.01). ns not significantly different.eChlorophyll content (A, B and total) of SD grown rosette leaves from Col-0,not4aand two independent complementation lines (N4A-G1andG3). Error bars = ±Standard Deviation.n= 5 biologically independent samples per genotype. Letters indicate one-way ANOVA; Tukey’s test (p< 0.05).fLugol’s iodine staining of Col-0 andnot4arosette leaves. Bar = 1 cm.gHistochemical staining of 7-day-old seedlings of theN4A-G3complementation line showing localisation ofpNOT4::NOT4-GUSto the first true leaves. This correlates with where the pale-yellow phenotype first presents innot4a(arrowhead) relative to Col-0. Bar = 200 µm. Images are representative of >10 independent seedlings.hDetection ofpNOT4::NOT4A-GUSby anti-GUS western blot in total vs chloroplast-specific protein extracts. LHCA4 is a chloroplast enriched protein control. UGPase is a cytosol control showing efficacy of chloroplast enrichment. RBCL was used as a loading control, and blots were repeated at least three times with similar results. Chloroplast function requires the coordinated action of nuclear- and chloroplast-derived proteins, including several hundred nuclear-encoded pentatricopeptide repeat (PPR) proteins that regulate plastid mRNA metabolism. Despite their large number and importance, regulatory mechanisms controlling PPR expression are poorly understood. Here we show that the Arabidopsis NOT4A ubiquitin-ligase positively regulates the expression of PROTON GRADIENT REGULATION 3 (PGR3), a PPR protein required for translating several thylakoid-localised photosynthetic components and ribosome subunits within chloroplasts. Loss of NOT4A function leads to a strong depletion of cytochrome b 6 f and NAD(P)H dehydrogenase (NDH) complexes, as well as plastid 30 S ribosomes, which reduces mRNA translation and photosynthetic capacity, causing pale-yellow and slow-growth phenotypes. Quantitative transcriptome and proteome analysis of the not4a mutant reveal it lacks PGR3 expression, and that its molecular defects resemble those of a pgr3 mutant. Furthermore, we show that normal plastid function is restored to not4a through transgenic PGR3 expression. Our work identifies NOT4A as crucial for ensuring robust photosynthetic function during development and stress-response, through promoting PGR3 production and chloroplast translation. The synthesis of energy from the sun, photosynthesis, supports organic life on earth. Light harvesting in green plants takes place within the specialized chloroplast organelle, believed to have arisen from engulfment of a photosynthetic prokaryote by an ancestral eukaryotic cell [1] . Coevolution and merging of these organisms has resulted in nuclear and chloroplast genomes separated within cellular compartments. In land plants, the chloroplast genome comprises ~130 genes, yet chloroplasts contain around 3000 different proteins [2] . Consequently, chloroplast function requires expression not only of chloroplast encoded proteins, but a multitude of nuclear-encoded genes, which are imported into chloroplasts post-translationally. One such group of nuclear derived factors is the pentatricopeptide repeat domain (PPR) containing proteins. The PPR protein family has significantly expanded in plants (~450 in Arabidopsis, vs <10 in humans and yeast [3] ), and members are characterized by a 35-amino acid repeat sequence that facilitates RNA binding and enables them to provide critical gene expression control within chloroplasts and mitochondria [4] . Through binding to organellar RNAs, PPR proteins stabilize gene transcripts, facilitate post-transcriptional processing and promote translation of the encoded proteins [4] , [5] . While their function in the regulation of gene expression control within organelles has been described, including many of the RNA species to which they bind, little is known about how their expression is regulated prior to import. Precise, selective removal of proteins is essential to cellular development and response. In eukaryotes, proteins can be marked for degradation by the megacomplex protease known as the 26 S proteasome, following enzymatic attachment of a chain of ubiquitin molecules [6] . Ubiquitin attachment requires sequential enzyme activities: initial processing of pre-ubiquitin by deubiquitinating enzymes (DUBs), followed by bonding to an E1 activating enzyme, transfer to an E2 conjugating enzyme, and finally, conjugation to a substrate mediated by an E3 ligase enzyme [7] . Despite the absence of the ubiquitin proteasome system (UPS) within plastids, several ubiquitin E3 ligases mediating chloroplast proteostasis have been described. The Hsc70-interacting protein (CHIP) E3 ligase was shown to target pre-plastid proteins for degradation in a chloroplast import-defective mutant background, indicating that it is required for ensuring correct and complete targeting of proteins to this organelle [8] , [9] , [10] . A second E3 ligase, Plant U-box ubiquitin-ligase PUB4, regulates the degradation of oxidatively damaged chloroplasts (Chlorophagy), via ubiquitination of envelope proteins [11] . Finally, a system for chloroplast-associated protein degradation (CHLORAD) targets damaged components of the chloroplast transmembrane protein import machinery (TOC) [12] . CHLORAD-targeted TOC subunits are ubiquitinated by the integral chloroplast outer membrane ubiquitin-ligase SP1, promoting removal and delivery to the 26 S proteasome via the mp85-type beta-barrel channel SP2 and AAA + chaperone CDC48 [12] , [13] , [14] . In addition, the 26 S proteasome was recently shown to counter-balance protein import into chloroplasts, with proteasome inhibition leading to enhanced import, and partial rescue of the TOC19a import mutant ( ppi2 ) through the introduction of mutations within proteasome subunits [15] . However, despite the evolutionary expansion and significance of the UPS in plants (accounting for more than 5% of the genome in Arabidopsis [16] ) the full extent to which the UPS can influence chloroplast function remains to be determined. The E3 ubiquitin-ligase NOT4 contains a unique combination of RING finger and RNA Recognition Motif (RRM) domains, which places its function at the interface of proteolysis and RNA biology [17] , [18] , [19] . Studies of NOT4 in yeast and animals have revealed that it associates with ribosomes, and plays a role in co-translational quality control of mRNA and protein, to ensure efficient and correct translation of polypeptides [17] , [20] , [21] , [22] , [23] . Furthermore, NOT4 regulates assembly and integrity of functional proteasomes in yeast [24] . Although it can exist as a monomer, NOT4 contributes to global RNA metabolism and gene expression control as a member of the CCR4-NOT complex [25] , [26] . While the NOT4 CCR4-NOT association is strong in yeast, structural and biochemical studies indicate it is more labile in animals, suggesting that general functions in translational regulation are conserved, but with kingdom-specific divergence in mechanism [27] , [28] . NOT4 has also been proposed to function as an N-recognin E3 ligase of the acetylation-dependent N-degron pathway in yeast [29] . Despite a central role for yeast and mammalian NOT4 in co-translational control and moderating the stabilities of mRNA and proteins, the presence and functions of NOT4-like E3 ligases in plants has not been investigated in detail previously. Here we identify three NOT4-like E3 ligases in Arabidopsis thaliana , and show that one of these—NOT4A—has diverged towards a key role in regulating chloroplast protein synthesis and photosynthetic function. We show that NOT4A is required for expression of the PPR protein PGR3, a nuclear-encoded factor that is imported into plastids to promote cytochrome b 6 f and NDH complex production, and ribosome biogenesis [30] , [31] , [32] , [33] . not4a mutants, which have severely depleted PGR3 levels, resemble null pgr3 mutants, having reduced abundance of plastid RNAs that are normally targeted by PGR3 and a depletion of 30 S ribosomes. There are also concomitant defects in chloroplast protein translation leading to to a pale-yellow phenotype, high-light stress sensitivity and compromised photosynthetic capacity. Site directed mutational analysis of NOT4A reveals its E3 ligase and RNA-binding functions are both essential to its chloroplast-related function, and transgenic expression of PGR3 in not4 a is sufficient to restore wild-type-like growth and development. Our work identifies NOT4A as an important mediator of PPR controlled plastid translation, uncovering a new layer of homeostatic and stress-responsive regulation controlling chloroplast form and function. Identification of NOT4-like proteins in Arabidopsis To identify NOT4-like proteins in plants we searched for protein sequences with homology to Sc NOT4 from Saccharomyces cerevisiae . In contrast to the single NOT4 gene present in humans, Drosophila and yeast, we identified three putative homologues in the model plant Arabidopsis thaliana , which we confirmed with reciprocal BLASTs. The three homologues, which we named NOT4A, -B and -C (AT5G60170, AT3G45630 and AT2G28540, respectively), possess 38–39% identity with Sc NOT4 (Fig. 1a and Supplementary Fig. 1 ), and crucially share high identity across the unique combination of RING, RRM and C3H1 domains. We isolated homozygous T-DNA insertion lines for NOT4A-C from publicly available collections (GABI-KAT, SALK and SAIL) and confirmed T-DNA inserts and full-length mRNA knockout (Supplementary Fig. 2A, B ). The not4a line displayed a pale-yellow phenotype and a clear delay in development, flowering significantly later than wild-type under normal growth conditions (Fig. 1b, d ). Moreover, the rosette leaves of not4a had a significant reduction of chlorophyll (Fig. 1e ), and Lugol’s staining revealed reduced starch accumulation relative to Col-0 in 6-week-old short-day grown plants (Fig. 1f ). In contrast, not4b and not4c displayed no obvious growth phenotypes, and so we decided to focus our attention on NOT4A. Fig. 1: Identification of NOT4-like proteins in Arabidopsis. a Schematic diagram of protein domain structure and % amino acid identity for Sachharomyces cerevisiae ( Sc ) and Arabidopsis thaliana ( At ) NOT4 proteins. For full sequence alignments see Supplementary Fig. 1 . b , c Representative rosette images of 4-week-old col-0, not4a-c mutants, and two independent not4a complementation lines ( N4A-G1 and G3 ) grown under long day (LD) conditions. Bar = 1 cm. d Days to flowering and rosette leaf number at flowering for genotypes shown under short-day (SD) conditions ( n = 10–12 per genotype). Box and whiskers plots show max and min, 25–75th percentiles (box), median (line) and mean (+). Letters indicate one-way ANOVA; Tukey’s test ( p < 0.01). ns not significantly different. e Chlorophyll content (A, B and total) of SD grown rosette leaves from Col-0, not4a and two independent complementation lines ( N4A-G1 and G3 ). Error bars = ±Standard Deviation. n = 5 biologically independent samples per genotype. Letters indicate one-way ANOVA; Tukey’s test ( p < 0.05). f Lugol’s iodine staining of Col-0 and not4a rosette leaves. Bar = 1 cm. g Histochemical staining of 7-day-old seedlings of the N4A-G3 complementation line showing localisation of pNOT4::NOT4-GUS to the first true leaves. This correlates with where the pale-yellow phenotype first presents in not4a (arrowhead) relative to Col-0. Bar = 200 µm. Images are representative of >10 independent seedlings. h Detection of pNOT4::NOT4A-GUS by anti-GUS western blot in total vs chloroplast-specific protein extracts. LHCA4 is a chloroplast enriched protein control. UGPase is a cytosol control showing efficacy of chloroplast enrichment. RBCL was used as a loading control, and blots were repeated at least three times with similar results. Full size image To confirm the pale-yellow not4a phenotype was due to loss of NOT4A expression we complemented the mutant by reintroduction of full-length genomic NOT4A with a c-terminal GUS tag, driven by ~2 kb of its endogenous promoter. Two independent transgenic lines expressing the full-length NOT4A protein (N4A-G1 and N4A-G3, Supplementary Fig. 2C ), displayed wild-type greenness and normal development (Fig. 1c–e ), and NOT4A expression, determined by GUS staining, was localized to the first true leaves of seedlings where the pale mutant phenotype first presents (Fig. 1g ). Analysis of the full-length NOT4A amino acid sequence using TargetP [34] revealed no obvious chloroplast transit peptide (cTP). In accordance with this prediction, anti-GUS western blotting of total vs chloroplast-specific protein extracts indeed revealed that NOT4A is not associated with this organelle, which is also in-line with the reported absence of the ubiquitin proteasome system in plastids (Fig. 1h ). NOT4A is required for normal photosynthetic function The growth, development and starch depletion phenotypes of not4a point to general defects in photosynthesis. To investigate this further, we carried out an RNA-seq analysis on 10-day-old not4a and Col-0 seedlings. This revealed a large number of differentially expressed genes (DEGs) in the mutant relative to WT (>2300 genes, P < 0.05), with GO-analysis showing that a large proportion of these are chloroplast-related and implicated across all structures of this organelle (Fig. 2a, b , Supplementary Fig. 3 and Supplementary Data 1 ). Carbon assimilation in stroma is undertaken by an array of higher order enzymatic complexes present within the internal membrane system of chloroplasts (thylakoids), which includes many nuclear-encoded components that were mis-regulated in the not4a transcriptome (Supplementary Fig. 3 and Supplementary Data 2 ) [35] . We therefore analysed the composition of the protein complexes within the thylakoids of Col-0, not4a and N4A-G3 complementation lines by blue native gel analysis (BN-PAGE) [36] , [37] , [38] . This revealed in not4a a severe decrease in the accumulation of protein bands corresponding to the photosystem II monomer and cytochrome b 6 f complex (PSII m/ Cyt b 6 f), as well as the photosystem I - NAD(P)H dehydrogenase megacomplex (PSI-NDH), when equal protein was loaded (Fig. 2c and Supplementary Fig. 4A ). Individual subunits were then resolved by a second denaturing dimension, which confirmed lower abundance of the PetA, -B, -C and -D cytochrome b 6 f complex subunits (Fig. 2d and Supplementary Fig. 4B ). Western blotting of total protein extracts further corroborated reduced abundance of PetC and NdhH, representative subunits of the cytochrome b 6 f and NDH complexes, in not4a (Fig. 2e ). In addition, dual-PAM measurements revealed a clear reduction in electron transfer rate (ETR) in not4a , consistent with depletion of cytochrome b 6 f within the thylakoid membranes (Fig. 2f ) [39] . Fig. 2: NOT4A is required for normal photosynthetic function. a Volcano plot of up and down DEGs in not4a vs WT. The top 8 DEGs are labelled (UP: AT5G44925, QQS/AT3G30720 and DOWN: AT4G13575, AT4G09875, AT3G10430, AT4G13572, PILS7/AT5G65980, UNE15/AT4G13560). b Graphical representation of ‘cell part’ and ‘chloroplast’ Gene Ontology (GO) enrichment of DEGs in not4a vs WT. Asterisk refers to significant enrichment; Fisher’s exact test, p < 0.001. c Blue native (BN) gel of thylakoid protein complexes from Col-0, not4a and N4A-G3 . Plants were grown under standard conditions (100 µmol photons m −2 s −1 , 8 h/16 h light/dark), and the entire thylakoid network was solubilized with 1% (w/v) dodecyl maltoside (DM) and separated using BN gel electrophoresis. 50 µg of total protein was loaded. Red and blue arrows refer to PSII m/Cyt b 6 f and PSI-NDH mc bands, respectively, which are significantly depleted in not4a . See also Supplementary Fig. 4A . d Second dimension separation of DM-solubilised thylakoid proteins from Col-0 and not4a showing depletion of cytochrome b 6 f components PetA, PetB, PetC and PetD in not4a . The protein bands were identified based on Aro et al. 2005 [36] . e Western blot determination of relative protein abundance of NdhH and PetC subunits of the NDH and cytochrome b 6 f complexes in Col-0 and not4a , with coomassie blue (CBB) staining to show comparable protein loading. f Light-intensity dependence of ETR(I) and ETR(II). Dark-adapted Col-0 and not4a plants were subjected to illumination steps of 3 min at light intensities of 25–1000 μmol photons m −2 s −1 followed by a saturating flash (700 ms) to determine F M’ and P M’ . The relative rates of electron transfer through PSI and PSII, ETR(I) and ETR (II), respectively, were calculated as Y(I) × PPFD × 0.84 × 0.5 and Y(II) × PPFD × 0.84 × 0.5. Each point represents the average ±SD ( n = 5 biological replicates). Gels and blots in Fig. 2c–e were repeated at least three times with similar results. Full size image NOT4A is required for plastid ribosome biogenesis To complement our RNA-seq analysis and investigate differences in protein abundance in not4a vs WT in more detail, we carried out a quantitative proteomics analysis of total protein extracts from 30-day-old whole plants as previously described [40] (Fig. 3a , Supplementary Data 2 ). Analysis of the chloroplast-specific proteins in these datasets (619 in WT, 689 in not4a; Fig. 3b ) confirmed reduced levels of all detected subunits making up the cytochrome b 6 f and NDH complexes, but also revealed that components of many other plastid enzyme complexes were mis-regulated (either increased or decreased in abundance) (Supplementary Fig. 4C and Supplementary Data 2 ). Fig. 3: NOT4A is required for plastid ribosome biogenesis. a , b Volcano plots showing differential abundance of total and plastid-localised proteins in not4a vs wild-type (Col-0) 30-day old-rosettes: x -axis, log2-Fold Change values of protein abundances in not4a versus wild-type; y -axis, log10-p values from a two-sided t -test. For the plastid-specific graph, photosynthetic and plastid ribosome proteins are highlighted in green and blue, respectively. The number of quantified proteins and their overlap are shown in Venn diagrams above each plot. The top 8 differentially accumulated proteins are labelled (UP: ALDH2C4/AT3G24503, VHA-E3/AT1G64200, HCF101/AT3G24430, AT2G42170, NS1/AT4G17300 and DOWN: AT3G47070, RPS2/ ATCG00160, ADK2/AT5G03300). c Histogram of summed protein amounts (ppm) of MapMan [90] annotated functional groups. Asterisk highlights 30 S ribosome group that is significantly depleted in not4a vs Col-0. Error bars = ±SEM. n = 3 biological replicates. p = 3.33E-08, students t -test, two tailed. d Western blot determination of relative protein abundance of 30 S subunits (RPS1 and RPS7) and 50 S subunits (RPL2 and RPL4) in Col-0 and not4a , with coomassie blue (CBB) staining to show comparable protein loading. Blots were repeated at least three times with similar results. e Relative amounts (ng/µl) of 50 S (23 s and 23 sb) and 30 S (16 s) plastid rRNAs in not4a vs Col-0. Values are quantified from Tapestation data shown in Supplementary Fig. 5, following normalisation to cytosolic 18 s rRNA. Error bars = ±SEM. n = 3 independent biological replicates. * p = 0.0446, ** p = 0.0037, students t -test, two tailed. f Heatmap showing relative transcript and protein fold-changes for 50 S and 30 S plastid ribosome subunits in not4a vs Col-0 (from RNA-seq and proteomics data). Red arrows denote subunits protein abundances confirmed by western blotting in d . See also Supplementary Data 2 . Full size image In addition to a reduction of photosynthetic proteins, we also observed a significant downregulation or absence of plastid ribosome proteins in not4a (Fig. 3b, f and Supplementary Data 2 ). This effect was specific to proteins making up the 30 S subunit of the chloroplast ribosome, while components of the 50 S subunit were detected at similar or slightly increased levels relative to wild-type (Fig. 3c, f ). Of twenty 30 S subunits identified in the proteomic analysis, 18 were significantly downregulated (>1.5 fold) in not4a vs WT, while none of the twenty six 50 S subunits identified were reduced in abundance. Western blotting corroborated the proteomics data, showing reduced levels of the 30 S subunits RPS1 and RPS7, no obvious change in the 50 S subunit RPL2, and slightly increased levels of the 50 S RPL4 protein in not4a (Fig. 3d ). We also observed a significant reduction of chloroplast 30 S-associated 16 S rRNA in not4a relative to WT, while levels of the 50 S-associated 23 S and 23 Sb rRNAs were similar or slightly increased (Fig. 3e and Supplementary Fig. 5 ). The reduction of 30 S subunits was only apparent at the protein level, as transcripts of the nuclear-encoded subunits were in fact elevated in the RNA-seq data (Fig. 3f , Supplementary Data 2 ). This indicates that decreased 30 S ribosome abundance in not4a is linked to a translational or post-translational, rather than transcriptional, defect. Plastid mRNA translation is compromised in the not4a mutant The reduction of 30 S ribosome subunits in not4a prompted us to investigate chloroplast translation in this mutant. We observed extreme hypersensitivity of not4a to the chloroplast ribosome-specific inhibitor lincomycin (Fig. 4a, b ). Lincomycin treated Col-0 seedlings were smaller in size and more yellow than control plants, resembling untreated not4a mutants, corroborating the observation that chloroplast ribosome activity is perturbed in not4a (Fig. 4a, b ). In contrast, no obvious differences in the sensitivity to the cytosolic ribosome inhibitor cycloheximide were observed (Supplementary Fig. 6A ). Next we assessed chloroplast-specific protein synthesis in WT and not4a by assaying incorporation rates of the aminoacyl-tRNA analogue puromycin into nascent proteins within isolated chloroplasts [41] . Puromycin-specific immunoblotting revealed a strong reduction of labelled proteins in not4a relative to WT, demonstrating reduced translational capacity in chloroplasts of the mutant (Fig. 4c ). Alongside the lincomycin results, this indicates that the reduced level of 30 S ribosomes in not4a causes defects in chloroplast mRNA translation. Fig. 4: Plastid mRNA translation is compromised in the not4a mutant. a 10-day-old WT, not4a and N4A-G3 seedlings grown on vertical plates ±10 µM lincomycin. Bar = 1 cm. b same as in a but on horizontal plates. Bar = 1 cm. c Protein synthesis rates in Col-0 and not4a chloroplasts, determined by anti-puromycin (α-Pur) western blot following a 2-h puromycin treatment time course. LHCA4 and CBB (Coomassie Brilliant blue) are shown as loading controls. Experiment was repeated at least three times with similar results. d The amount of D1 protein (% of 0 h) and PSII efficiency (F V /F M ) during a photoinhibitory treatment at 1000 μmol photons m −2 s −1 with and without lincomycin (linc) and during recovery without linc at 100 μmol photons m −2 s −1 . Total leaf protein extracts were separated on an SDS-PAGE, immunoblotted with a D1-specific antibody and quantified with LI-COR imaging. Averages from three biological replicates are presented with ±SEM error bars. Source data are included in the Source Data file. e Quantitative RT-PCR (qPCR) of NOT4A in 14-day-old Col-0 lines grown on media ±10 µM Lincomycin. Expression levels normalised to ACTIN7 and shown relative to untreated Col-0. Averages from three biological replicates are presented with ±SEM error bars. Full size image To explore these translational defects further we focussed on chloroplast encoded D1, a photolabile protein that is enzymatically broken down after light-induced damage [42] . The high turnover rate of the D1 protein requires rapid synthesis and replacement to reassemble the PSII complex, which is essential for photosynthesis. We examined D1 turnover and PSII efficiency before, during and after high light (HL) exposure in not4a and Col-0 plants. Comparable levels of D1 in not4a and Col-0 before HL stress suggests sufficient basal translation under nonstressed conditions, despite reduced ribosome abundance (Fig. 4d and Soure Data). After 1.5 h of HL D1 was reduced to <50% of starting levels in not4a , whereas levels in Col-0 were maintained above 80%. This is in-line with the detected PSII activities, measured as F v /F M , which decreased in both lines, but less severely in Col-0. After 16 h of recovery in standard conditions (GL), Col-0 D1 levels returned to nearly 100%, while in not4a they remained below 55%, implying defects in D1 biosynthesis. Reduction of D1 when lincomycin was applied during HL treatment to inhibit translation confirmed that D1 synthesis compensates for damaged and degraded protein in Col-0. Thus, reduced abundance of plastid ribosomes in not4a leads to severely reduced translational capacity in response to stress. We also found that NOT4A expression was upregulated when seedlings were grown in the presence of lincomycin, suggesting NOT4A expression is controlled by plastid-to-nucleus retrograde signalling during chloroplast translational stress (Fig. 4e ). Taken together these data show that NOT4A is required to maintain homeostatic and stress-responsive translational productivity in chloroplasts. Functional domain analysis of NOT4A To investigate the mechanistic connection between NOT4A and chloroplast function in more detail, we mutated the conserved RING and RRM domains in pNOT4A::NOT4A-GUS and tested if these variants could still complement the not4a mutant. These mutations were based on conserved homologies to yeast Sc NOT4 where the activities of both domains were successfully knocked out previously (Fig. 5a and Supplementary Fig. 1 ) [18] , [23] , [43] . NOT4A proteins containing either a single L11A mutation in the N-terminal RING domain, three point mutations in the RRM domain (G137A, Y166A and C208A), or all four substitutions were expressed under the endogenous promoter (Fig. 5b ). We observed particularly high levels of the L11A RING mutant variant, suggesting that abolishing RING activity may enhance NOT4A stability by preventing auto-ubiquitination, a common feature in E3 ubiquitin-ligase regulation [44] . Mutation of the RRM, however, resulted in reduced NOT4A levels, potentially due to disruption of protein activity leading to enhanced auto-ubiquitination, a notion supported by comparatively increased abundance of combined RING/RRM mutations. In contrast to complementation with WT pNOT4A::NOT4A-GUS , none of the mutant variants were functional in planta, as evidenced by the incapacity to restore WT tolerance to lincomycin or revert the pale-yellow phenotype of the not4a mutant (Fig. 5c, d ). Overall, we can deduce that both domains of NOT4A are required for its role in regulating chloroplast function. Fig. 5: Functional domain analysis of NOT4A. a Schematic diagram showing position of point mutations in RING and RRM domains. Mutations in black are those introduced to the NOT4A gene, which correspond to equivalent conserved residues in Sc NOT4 (shown in grey), additionally highlighted in Supplementary Fig. 1 sequence alignments. b anti-GUS western blot of steady state levels of pNOT4A::NOT4A -GUS variants expressed in not4a . Blots were repeated at least three times with similar results. c 10-day-old not4a and pNOT4A::NOT4A -GUS complementation lines grown on vertical plates ±10 µM lincomycin. Bar = 1 cm. d Representative rosette images of 3-week-old not4a and pNOT4A::NOT4A -GUS complementation lines under long day (LD) conditions. Bar = 1 cm. Full size image The not4a mutant mimics the pgr3 mutant To identify potential causal agents of the phenotypic defects in not4a we analysed the DEGs annotated with chloroplast functions (GO:0009507) in the not4a RNA-seq dataset (Fig. 6a , Supplementary Data 1 ). A total of 819 DEGs were identified, with a vast majority of these (693) being upregulated relative to WT. Amongst these genes were 34 chloroplast-targeted PPR proteins, which collectively may be upregulated to compensate for compromised chloroplast translation in the mutant (Supplementary Fig. 6B , Supplementary Data 2 ) [45] , [46] , [47] . Interestingly, we found that mRNA encoding one of these chloroplast-targeted PPR proteins, PROTON GRADIENT REGULATION 3 (PGR3) (AT4G31850), was downregulated to undetectable levels in not4a , but restored to WT levels in the N4A-G3 complementation line (Fig. 6b and Supplementary Fig. 6B ). PGR3 was originally identified in a screen for mutants with defects in nonphotochemical quenching (NPQ) determined by chlorophyll fluorescence [30] . The compromised NPQ and ETR of pgr3 mutants was subsequently attributed to PGR3′s role in promoting stabilisation and translation of the chloroplast PetL operon (which encodes for the cytochrome b 6 f subunits PetL and PetG), as well as a role in regulating production of the NDH subunit NdhA. As such, pgr3 mutants have reduced levels of cytochrome b 6 f and NDH, similar to not4a (Fig. 2c–e and Supplementary Fig. 4A, B, D ) [30] , [31] , [32] , [33] . Moreover, pgr3 mutants in maize were shown to have reduced levels of chloroplast ribosomes, which also resembles our observations in not4a [48] . Fig. 6: The not4a mutant mimics the pgr3 pentatricopeptide mutant. a Volcano plot of GO chloroplast-associated (GO:0009507) DEGs in not4a vs WT. The top 8 DEGs are labelled (UP: ELIP2/AT4G14690, ELIP1/AT3G22840, PGL5/AT5G24420 and DOWN: AT3G55240, AT5G24240, SAUR1/AT4G34770, PLP2/AT2G26560, AT4G16620). b Quantitative PCR (qPCR) of PGR3 in Col-0, not4a and N4A-G3 complementation line. Expression levels normalised to ACTIN7 and shown relative to Col-0 WT. Error bars = ±SEM. n = 3 biological replicates. Letters indicate one-way ANOVA; Tukey’s test ( p < 0.01). c Representative rosette images of 4-week-old Col-0, not4a , Ws-4 and pgr3-4 lines grown under long day (LD) conditions. Bar = 1 cm. d 10-day-old Col-0, not4a , Ws-4 and pgr3-4 seedlings grown on vertical and horizontal plates ±10 µM lincomycin. Bar = 1 cm. e Western blot determination of 30 S ribosome subunits (RPS1 and RPS7), 50 S ribosome subunits (RPL2 and RPL4), PetC and NdhH in Col-0, not4a , Ws-4 and pgr3-4 with coomassie blue (CBB) staining to show comparable protein loading. Blots were repeated at least three times with similar results. f qPCR of PetL and PetG in 10-day old Col-0, not4a , Ws-4 and pgr3-4 seedlings. Expression levels normalised to ACTIN7 and shown relative to Col-0 WT. Data are average of three biological replicates. Letters indicate one-way ANOVA; Tukey’s test ( p < 0.01). Error bars = ±SEM. g Relative amounts (ng/μl) of 50 S (23 s and 23 sb) and 30 S (16 s) plastid rRNAs in Col-0, not4a , Ws-4 and pgr3-4 seedlings. Values are quantified from Tapestation data shown in Supplementary Fig. 5 , following normalisation to cytosolic 18 s rRNA. Col-0 and not4a data are same as in Fig. 3e . Error bars = ±SEM. n = 3 biological replicates. * p = 0.0446, ** p = 0.0037, *** p = 0.027, students t -test, two-tailed. h ETR(I) and ETR(II) during an induction curve measurement. Dark-adapted Col-0, not4a , Ws-4 and pgr3 plants were illuminated with 1000 μmol photons m −2 s −1 actinic light and a saturating flash was applied every 2 min to determine F M’ and P M’ . The relative rates of electron transfer through PSI and PSII, ETR(I) and ETR (II), respectively, were calculated as in Fig. 2 . Each point represents the average ±SD ( n = 3–4). Full size image We acquired a recently isolated null mutant of PGR3 in the Arabidopsis Wassilewskija-4 (Ws-4) ecotype, pgr3-4 [33] , and showed that this shares a similar delayed development and pale-yellow phenotype with not4a (Fig. 6c ). Reduced transcripts of PetL and PetG , but not PetA , B and D , were detected in both not4a and pgr3-4 relative to their respective wildtypes, consistent with the requirement for PGR3 in stabilising these two RNAs (Fig. 6f and Supplementary Fig. 6C, D ). The reduced abundance of PetC and NdhH proteins seen in not4a was also observed in pgr3-4 (Fig. 6e ) [30] , [31] , [32] , [33] , and both mutants had a similar reduction in ETR (Fig. 6h ). In contrast, steady state protein levels of the Rubisco subunit RBCL, PSII subunits D1 and PsbP, and the PSI-associated protein LHCA4 were not significantly altered relative to WT in either mutant under nonstressed conditions (Supplementary Fig. 4E ). To determine if PGR3 plays a role in general chloroplast translation like NOT4A, we tested sensitivity of the mutant to lincomycin. Here, pgr3-4 displayed a similar degree of hypersensitivity as not4a (Fig. 6d ) . Our proteomic data indicated that the lincomycin sensitivity of not4a is likely due to depletion of the 30 S subunit of chloroplast ribosomes in the mutant (Fig. 3 ). Like not4a , the pgr3-4 mutant had reduced abundance of 30 S chloroplast ribosome subunits RPS1 and RPS7, while levels of the 50S RPL2 and RPL4 subunits were comparable to WT (Fig. 6e ). Furthermore, there is a significant reduction in the 30 S associated 16 S rRNA in both mutants (Fig. 6g and Supplementary Fig. 5 ). Collectively, these data demonstrate a comparable depletion of the cytochrome b 6 f complex, NDH complex, and 30 S chloroplast ribosome in not4a and pgr3-4 . In Arabidopsis, PGR3 was recently shown to control stability and stimulate expression of the 30 S Rps8 and 50 S Rpl14 ribosomal subunits [33] , revealing a key role for this protein in promoting ribosome biogenesis. Interestingly a second PPR protein, SVR7, also regulates Rpl14 stability, but does not affect Rps8 translation [33] , [49] . 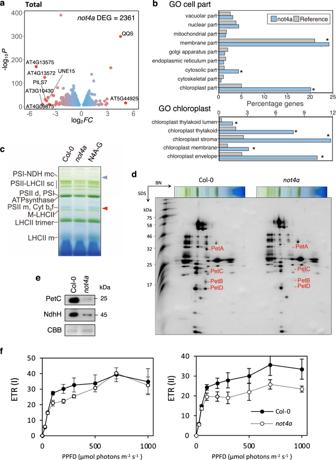Fig. 2: NOT4A is required for normal photosynthetic function. aVolcano plot of up and down DEGs innot4avs WT. The top 8 DEGs are labelled (UP: AT5G44925, QQS/AT3G30720 and DOWN: AT4G13575, AT4G09875, AT3G10430, AT4G13572, PILS7/AT5G65980, UNE15/AT4G13560).bGraphical representation of ‘cell part’ and ‘chloroplast’ Gene Ontology (GO) enrichment of DEGs innot4avs WT. Asterisk refers to significant enrichment; Fisher’s exact test,p< 0.001.cBlue native (BN) gel of thylakoid protein complexes from Col-0,not4aandN4A-G3. Plants were grown under standard conditions (100 µmol photons m−2s−1, 8 h/16 h light/dark), and the entire thylakoid network was solubilized with 1% (w/v) dodecyl maltoside (DM) and separated using BN gel electrophoresis. 50 µg of total protein was loaded. Red and blue arrows refer to PSII m/Cyt b6f and PSI-NDH mc bands, respectively, which are significantly depleted innot4a. See also Supplementary Fig.4A.dSecond dimension separation of DM-solubilised thylakoid proteins from Col-0 andnot4ashowing depletion of cytochrome b6f components PetA, PetB, PetC and PetD innot4a. The protein bands were identified based on Aro et al. 200536.eWestern blot determination of relative protein abundance of NdhH and PetC subunits of the NDH and cytochrome b6f complexes in Col-0 andnot4a, with coomassie blue (CBB) staining to show comparable protein loading.fLight-intensity dependence of ETR(I) and ETR(II). Dark-adapted Col-0 andnot4aplants were subjected to illumination steps of 3 min at light intensities of 25–1000 μmol photons m−2s−1followed by a saturating flash (700 ms) to determine FM’and PM’. The relative rates of electron transfer through PSI and PSII, ETR(I) and ETR (II), respectively, were calculated as Y(I) × PPFD × 0.84 × 0.5 and Y(II) × PPFD × 0.84 × 0.5. Each point represents the average ±SD (n= 5 biological replicates). Gels and blots in Fig.2c–ewere repeated at least three times with similar results. We observed enhanced levels of SVR7 protein in not4a relative to WT (Supplementary Fig. 6B ), perhaps compensating for loss of PGR3 , and explaining why 50 S subunits are not affected in the mutant. Defects in Rps8 translation due to loss of PGR3 in not4a may explain why ribosome depletion is specific to the 30 S subunit, since protein complex stoichiometries are highly regulated, with the inability to assemble complete complexes often leading to degradation of orphan subunits [50] , [51] . The upregulation of PPR proteins SOT1, EMB2654, PPR4 and PPR2 (which all promote chloroplast rRNA maturation), and GUN1 (implicated in the production of chloroplast ribosomal subunits RPS1 and RPL11) present further evidence of compensatory responses to reduced ribosome abundance and protein synthesis within not4a chloroplasts (Supplementary Fig. 6B ) [52] , [53] , [54] , [55] , [56] . PGR3 can rescue the chloroplast-associated defects in not4a Our data indicate that the not4a defects in chloroplast ribosome abundance, protein translation and photosynthetic function may be linked to reduced PGR3 expression in this mutant. We therefore investigated the effect of ectopic PGR3 e xpression on not4a phenotypes by transforming not4a and Col-0 with a functional pPGR3::PGR3-YFP construct capable of complementing pgr3-4 (Supplementary Fig. 7a ). PGR3-YFP protein levels were comparable across the Col-0 and not4a lines, while PGR3 transcripts were elevated between 2- and 6-fold above WT levels in all transgenics, with YFP- specific qPCR corroborating the proportional pattern of expression between lines (Fig. 7a, b and Supplementary Fig. 7B ). When compared to their untransformed backgrounds, two of the three Col-0 (lines 1 and 2) and all not4a lines, possessed higher transcript levels than attributable to the doubled PGR3 gene copy number present in homozygous transgenics, suggesting a decoupling from endogenous negative regulation (Fig. 7b ). Fig. 7: PGR3 can rescue the chloroplast-associated defects in not4a . a Anti-YFP western blot of steady state PGR3-YFP protein levels in three independent Col-0 and not4a lines expressing pPGR3::PGR3-YFP . b Quantitative PCR (qPCR) of PGR3 in Col-0, not4a and the PGR3-YFP lines from a . Expression levels normalised to ACTIN7 and shown relative to Col-0 WT. n = 3 biological replicates. Error bars = SEM. c Confocal images of hypocotyl cells in Col-0 and not4a lines expressing pPGR3::PGR3-YFP . Panels show PGR3-YFP in green (left), chloroplasts in red (middle) and bright field view (right). Experiment was replicated at least 3 times (see Supplementary Fig. 7D for further repeats). d 10-day-old Col-0, not4a and PGR3-YFP transgenic seedlings grown on vertical plates ±10 µM lincomycin. Bar = 1 cm. e Representative rosette images of 4-week-old Col-0, not4a and not4a PGR3-YFP lines grown under long day (LD) conditions. Bar = 1 cm. f Cycloheximide (CHX) chase of PGR3-YFP and ACTIN in Col-0 and not4a ± bortezomib (BZ). g Yeast two-hybrid assay between NOT4A and PGR3. EV empty vector. P53/SV40 positive control. Growth on -LW confirms successful transformation; growth on -AHLW denotes interaction. Western blots in 7a and 7f were repeated three times with similar results. Full size image PGR3-YFP localized as expected within chloroplasts in both backgrounds (Fig. 7c and Supplementary Fig. 7D ). Given that the NOT4A RING mutant is nonfunctional in Arabidopsis (Fig. 5 ) and NOT4 ubiquitin E3 ligase activity promotes proteasomal degradation of substrates in other organisms, we tested if NOT4A might target PGR3 to the UPS. Inhibition of protein synthesis using cycloheximide neither led to degradation of PGR3-YFP in WT or not4a lines, nor did proteasome inhibition with bortezomib (BZ) enhance its stability, indicating PGR3 is not a proteolytic target of NOT4A E3 ligase activity (Fig. 7f ). This is further supported by an inability to detect ubiquitin modification of immunoprecipitated PGR3-YFP (Supplementary Fig. 8 ) and an absence of a protein-protein interaction between NOT4A and PGR3 when assayed by yeast two-hybrid (Fig. 7g ). Remarkably however, introduction of the pPGR3::PGR3-YFP transgene was able to complement the pale-yellow and lincomycin-sensitive phenotypes of not4a , despite the lack of NOT4A expression (Fig. 7d, e and Supplementary Fig. 7C ). Given that we have shown it is possible to express functional PGR3 driven by its native promoter in the not4a mutant, we backcrossed not4a to WT Col-0 and reselected for the not4a mutation to ensure the endogenous PGR3 was not aberrant, and found that the not4a phenotype persisted in backcrossed plants when bred to homozygosity for the T-DNA insert. This, along with our prior observation that reintroduction of pNOT4A::NOT4A-GUS into not4a can restore PGR3 transcript levels (Figs. 1c , 4a , 6b ), indicates NOT4A is required for PGR3 expression and suggests that the inclusion of c-terminal YFP and/or a lack of regulatory elements in the reintroduced pPGR3::PGR3 construct decouples PGR3 regulation from NOT4A control in the mutant. This scenario is further supported by increased accumulation of PGR3 transcripts in the Col-0 and not4a pPGR3::PGR3 transgenic lines relative to WT (Fig. 7b ). As essential components of the gene expression machinery in plastids, nuclear-encoded PPR proteins must be dynamically controlled in order to meet the fluctuating demands of the light-harvesting chloroplast organelle. However, relatively little is known about how PPR proteins are regulated. Here we show that expression of PGR3, a large PPR protein that regulates chloroplast RNAs involved in cytochrome b 6 f/NDH complex formation and chloroplast ribosome biogenesis, is regulated by the cytosolic E3 ubiquitin-ligase NOT4A. We found that not4a mutants have photosynthetic and growth defects that are a consequence of highly reduced cytochrome b 6 f and NDH complexes, as well as 30 S ribosomal subunits. Transcripts encoding PGR3 are undetectable in not4a , and the pgr3-4 mutant shares functional defects in chloroplast translation and photosynthetic activity. The chloroplast-related defects of not4a can be restored by introducing PGR3-YFP expressed from the endogenous PGR3 promoter sequence. While the molecular connection between NOT4A and PGR3 remains to be defined, our work identifies a previously undescribed link between an evolutionarily conserved E3 ubiquitin-ligase, control of PPR protein expression and the regulation of chloroplast function. Our data suggest that PGR3 protein is not a direct proteolytic target of NOT4A. Based on known activities of NOT4 in yeast, Drosophila and mammals, we postulate instead that NOT4A is required to suppress negative regulation of PGR3 expression at regulatory sequences outside of the reintroduced PGR3-encoding transgene, such as the 3′ UTR or distal elements. This regulation could be direct, or could occur indirectly by controlling the transcript or protein stability of other factors that regulate PGR3. NOT4-like proteins are unique amongst E3 ubiquitin ligases, in that they consist of both a RING domain an RNA-binding RRM domain [19] . We showed that both these domains are required for the chloroplast-related functions of NOT4A hence presumably promotion of PGR3 expression. Although RNA-binding specificity is unknown, RNA-binding activities of NOT4B and NOT4C were previously observed in a proteome-wide survey of Arabidopsis RNA-binding proteins [57] . Mammalian NOT4 was found to bind stalled ribosome complexes undertaking co-translational import into damaged mitochondria, initiating quality control, and ultimately mitophagy [17] . While the repetitive domain structures of PPR proteins enable precise and selective RNA binding, they may also present a translational challenge to ribosomes. Two profiling studies of the Arabidopsis RNA degradome together identified five PPR genes as targets for co-translational mRNA decay, with further analysis identifying three nucleotide periodicity within one PRR transcript suggestive of ribosome stalling [58] , [59] . PGR3 is the second largest and most structurally repetitive (containing 25 repeats, determined by RADAR [60] ) of the 34 DEG chloroplast-targeted PPR genes in not4a . Hence, potential co-translational regulation of PGR3 transcripts by NOT4A warrants further investigation in plants. In other organisms NOT4 contributes to post-transcriptional control as a component of the CCR4-NOT complex, central to mRNA 3′ deadenylation, promotion of decapping and subsequent mRNA decay [25] , [26] . NOT4 in yeast was recently shown to be essential for the turnover of mRNAs with low codon optimality during translation, triggering recruitment of the CCR4-NOT complex through catalysing ribosome ubiquitination [61] . Although the presence of NOT4 within the CCR4-NOT complex in plants has yet to be established [62] , a recent proteomic characterisation of Target of rapamycin (TOR) signalling in Arabidopsis identified NOT4A as a TOR-regulated phosphoprotein, and NOT4B as an LST8 interactor along with other conserved CCR4-NOT core subunits, suggesting the plant NOT4s may indeed be subunits within this complex [63] . Furthermore, in humans and Drosophila, NOT4 contains a c-terminal sequence required for binding to the CCR4-NOT linker protein CAF40, and a similar sequence exists in Arabidopsis NOT4A [28] . Given the links between TOR, mRNA translation and plastid ribosome regulation [64] , [65] , the connection between TOR and NOT4A within the context of the CCR4-NOT complex requires exploration. Within the CCR4-NOT complex, the CAF1 subunit binds to the central NOT1 scaffold to provide deadenylase activity in humans and Drosophila [66] , [67] . The CAF1 family has expanded and diverged in plants, with only a proportion of members capable of binding NOT1, which are also able to bind with CCR4 to form a deadenylating module within the CCR4-NOT complex in Arabidopsis and rice [62] , [68] . It has been proposed that these differing binding activities of CAF1 proteins represent distinct assemblies of the CCR4-NOT complex [62] , highlighting the potential functional expansion of the complex in plants, which could be further increased via the three NOT4 homologues we have identified here. Exploring the in vivo targets of E3 ligase and RNA-binding activities of all three Arabidopsis NOT4 proteins, in addition to determining their association and function within the CCR4-NOT complex, will help to shed light not only on how NOT4A regulates PGR3 expression and chloroplast function, but also how these enigmatic E3 ubiquitin ligases influence other aspects of plant biology. Arabidopsis growth and transgenic lines Seed were sown on compost mixed to a ratio 4:2:1 of Levington F2 compost, vermiculite and perlite, or sterile half strength Murashige & Skoog (MS) medium with 0.8% agar made with purified water and autoclaved for 15 min at 121 °C. Plants were grown in Weiss Technik fitotron SGC 120 biological chambers with 16-h light/8-h dark cycles at 22 °C (long day), or 12-h light/ 12-h dark at 22 °C (short day). T-DNA insertion mutants were identified from the GABI-KAT ( not4a ; GABI_134E03) [69] , SAIL ( not4b ; SAIL_274_D03) [70] and SALK ( not4c ; SALK_093123) [71] , collections from the Nottingham Arabidopsis Stock Centre (NASC) and the pgr3-4 (line FLAG 086D06) from the Versailles Arabidopsis thaliana Stock Center [33] . Homozygous T-DNA insertions were identified by PCR with primers designed by T-DNA express and null expression confirmed by RT-PCR (Supplementary Fig. 2A, B ). 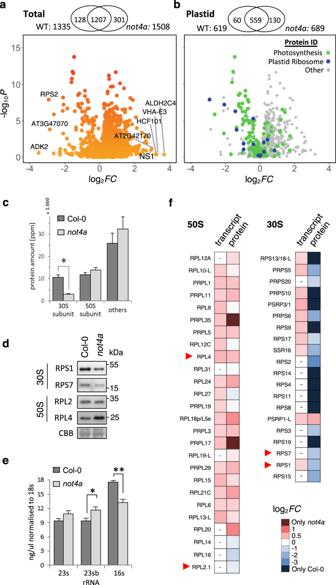Fig. 3: NOT4A is required for plastid ribosome biogenesis. a,bVolcano plots showing differential abundance of total and plastid-localised proteins innot4avs wild-type (Col-0) 30-day old-rosettes:x-axis, log2-Fold Change values of protein abundances innot4aversus wild-type;y-axis, log10-p values from a two-sidedt-test. For the plastid-specific graph, photosynthetic and plastid ribosome proteins are highlighted in green and blue, respectively. The number of quantified proteins and their overlap are shown in Venn diagrams above each plot. The top 8 differentially accumulated proteins are labelled (UP: ALDH2C4/AT3G24503, VHA-E3/AT1G64200, HCF101/AT3G24430, AT2G42170, NS1/AT4G17300 and DOWN: AT3G47070, RPS2/ ATCG00160, ADK2/AT5G03300).cHistogram of summed protein amounts (ppm) of MapMan90annotated functional groups. Asterisk highlights 30 S ribosome group that is significantly depleted innot4avs Col-0. Error bars = ±SEM.n= 3 biological replicates.p= 3.33E-08, studentst-test, two tailed.dWestern blot determination of relative protein abundance of 30 S subunits (RPS1 and RPS7) and 50 S subunits (RPL2 and RPL4) in Col-0 andnot4a, with coomassie blue (CBB) staining to show comparable protein loading. Blots were repeated at least three times with similar results.eRelative amounts (ng/µl) of 50 S (23 s and 23 sb) and 30 S (16 s) plastid rRNAs innot4avs Col-0. Values are quantified from Tapestation data shown in Supplementary Fig.5,following normalisation to cytosolic 18 s rRNA. Error bars = ±SEM.n= 3 independent biological replicates. *p= 0.0446, **p= 0.0037, studentst-test, two tailed.fHeatmap showing relative transcript and protein fold-changes for 50 S and 30 S plastid ribosome subunits innot4avs Col-0 (from RNA-seq and proteomics data). Red arrows denote subunits protein abundances confirmed by western blotting ind. See also Supplementary Data2. Arabidopsis lines were transformed with the genomic sequences of NOT4A (AT5G60170) and PGR3 (AT4G31850) plus ~2KB of the upstream promoters cloned into Invitrogen pENTR™/D-TOPO™ (ThermoFisher- K240020) (For primer sequences see Supplementary Data 3 ) and sequenced before ligations into pGWB533 and pGWB540 constructs respectively [72] , using the Agrobacterium tumefaciens (GV3101 pMP90) floral dip method [73] . Histochemical staining GUS staining was performed using 1% potassium ferricyanide and potassium ferrocyanide added to the GUS stain solution (0.1 M PBS, pH 7.0, 2 mM X-gluc and Triton-X-100 (0.1% v/v) [74] . Seedlings were submerged in 1 ml of GUS stain solution and were incubated at 37 °C in the dark for 24 h. GUS stain solution was replaced by 1 ml of fixative (3:1 ethanol:acetic acid, 1% Tween v/v). Samples were incubated at room temperature with gentle shaking and fixative refreshed until tissues appeared cleared. Cleared samples were then mounted onto microscope slides in 50% glycerol and images captured with a bifocal light microscope. Starch content was assessed using Lugol’s iodine staining of 6-week-old short-day grown rosette leaves as described [75] . Tissue was precleared with ethanol and washed in distilled water before adding Lugol’s solution with rocking at room temperature (6 mM iodine, 43 mM KI and 0.2 M HCl), this was then washed with distilled water until clear. Phenotypic assays Flowering time determined from 12 plants per line, grown under short and long day conditions. Plants were assessed daily, once a bolt of >1 cm was produced the number of rosette leaves and day number was recorded. Lincomycin sensitivity was assayed on half MS agar plates supplemented with 10 µM. Lincomycin hydrochloride monohydrate (VWR- ALEXBML-A240). Sterilised seed were plated and stratified for 48 h, then grown for 7–10 days with 16-h light/8-h dark cycles at 22 °C. Chlorophyll was quantified from 60 mg of frozen 6-week-old short-day grown rosette leaves. 1.8 ml of DMF at 4 °C was added and tubes inverted twice and incubated for 16 h at 4 °C. Absorbance was measured using BMG labtech FLUOstar OPTIMA spectrometer at 664.5 nm 647 nm for four biological replicates per line, chlorophyll content calculated as [76] . RNA-seq analysis RNA was extracted using Qiagen Plant RNAeasy extraction kit as per manufacturers guidelines. RNA degradation and contamination was monitored on 1% agarose gels. Transcriptome sequencing and analysis was performed by Novogene (UK) Company Limited, 25 Cambridge Science Park, Milton Road, Cambridge, CB4 0FW, United Kingdom. RNA purity was checked using the NanoPhotometer ® spectrophotometer (IMPLEN, CA, USA). RNA concentration was measured using Qubit ® RNA Assay Kit in Qubit® 2.0 Flurometer (Life Technologies, CA, USA). RNA integrity was assessed using the RNA Nano 6000 Assay Kit of the Bioanalyzer 2100 system (Agilent Technologies, CA, USA). A total amount of 3 μg RNA per sample was used as input material for the RNA sample preparations. Sequencing libraries were generated using NEBNext® UltraTM RNA Library Prep Kit for Illumina ® (NEB, USA) following manufacturer’s recommendations. mRNA was purified from total RNA using poly-T oligo-attached magnetic beads. Fragmentation was carried out using divalent cations under elevated temperature in NEBNext First Strand Synthesis Reaction Buffer(5X). First strand cDNA was synthesized using random hexamer primer and M-MuLV Reverse Transcriptase (RNase H - ). Second strand cDNA synthesis was subsequently performed using DNA Polymerase I and RNase H. Remaining overhangs were converted into blunt ends via exonuclease/polymerase activities. After adenylation of 3′ ends of DNA fragments, NEBNext Adaptor with hairpin loop structure were ligated to prepare for hybridization. In order to select cDNA fragments of preferentially 150~200 bp in length, the library fragments were purified with AMPure XP system (Beckman Coulter, Beverly, USA). Then 3 μl USER Enzyme (NEB, USA) was used with size-selected, adaptor-ligated cDNA at 37 °C for 15 min followed by 5 min at 95 °C before PCR. Then PCR was performed with Phusion High-Fidelity DNA polymerase, Universal PCR primers and Index (X) Primer. At last, PCR products were purified (AMPure XP system) and library quality was assessed on the Agilent Bioanalyzer 2100 system. The clustering of the index-coded samples was performed on a cBot Cluster Generation System using HiSeq PE Cluster Kit cBot-HS (Illumina) according to the manufacturer’s instructions. After cluster generation, the library preparations were sequenced on an Illumina Hiseq platform and 125 bp/150 bp paired-end reads were generated. Raw data (raw reads) of fastq format were firstly processed through in-house perl scripts. In this step, clean data (clean reads) were obtained by removing reads containing adapter, reads containing ploy-N and low quality reads from raw data. At the same time, Q20, Q30 and GC content the clean data were calculated. All the downstream analyses were conducted in R (R Core Team, 2014) based on the clean data with high quality and figures were produced using the package ggplot2 [77] . Reference genome and gene model annotation files were downloaded from genome website directly. Index of the reference genome was built using Bowtie v2.2.3 and paired-end clean reads were aligned to the reference genome using TopHat v2.0.12. We selected TopHat as the mapping tool for that TopHat can generate a database of splice junctions based on the gene model annotation file and thus a better mapping result than other nonsplice mapping tools. HTSeq v0.6.1 was used to count the reads numbers mapped to each gene. And then FPKM of each gene was calculated based on the length of the gene and reads count mapped to this gene. FPKM, expected number of Fragments Per Kilobase of transcript sequence per Millions base pairs sequenced, considers the effect of sequencing depth and gene length for the reads count at the same time, and is currently the most commonly used method for estimating gene expression levels [78] . Differential expression analysis for the not4a mutant compared to Col-0 (WT) (three biological replicates per genotype) was performed using the DESeq R package (1.18.0). DESeq provide statistical routines for determining differential expression in digital gene expression data using a model based on the negative binomial distribution [79] . The resulting P values were adjusted using the Benjamini and Hochberg’s approach for controlling the false discovery rate [80] . Genes with an adjusted P -value < 0.05 found by DESeq were assigned as differentially expressed. Gene Ontology (GO) enrichment analysis of differentially expressed genes was implemented using AgriGO [81] . Quantitative RT-PCR Arabidopsis seedlings were frozen in liquid nitrogen and ground to a fine powder. RNA was extracted using the Qiagen Plant RNAeasy kit as per manufacturers recommendations. RNA was quantified using a Thermo Scientific NanoDropTM 1000 Spectrophotometer. 1.5 µg of RNA was treated with RQ1 DNase (Promega- M6101) as per manufacturers recommendations. cDNA was synthesized using oligo dT or random hexamers (for analysis of chloroplast encoded petL and -G transcripts) and SuperScript® II Reverse Transcriptase. cDNA was assessed for genomic DNA contamination using intron spanning primers for ACTIN7 . Quantitative PCR primers were designed using the NCBI primer BLAST [82] and primer annealing was tested using gradient PCR. Relative expression was compared between genotypes and treatments using target primers and primers to the housekeeping gene ACTIN7 for normalization (For primer sequences see, Supplementary Data 3 ). Agilent Brilliant III SYBR was used in conjunction with Agilent Aria MX qPCR machine and analysis performed using the ∆∆CT comparative quantification method [83] . rRNA analysis Total RNA was extracted and quantified as described above and run on an Agilent Tapestation 2200. The concentration of RNA peaks of appropriate sizes corresponding to the abundant ribosomal RNAs (23 S, 23Sb, 18 S and 28 S) were determined with provided software normalized to a RNA ladder standard. As no differences in cytosolic ribosome abundance was observed in the mutants, 18 S rRNA was used to normalize chloroplast rRNA concentrations within samples to aid comparison between genotypes. Western blotting The BIORAD Mini PROTEAN system was used for gel casting, running and transfer. 10% polyacrylamide gels (resolving gel: 0.38 M tris-HCl pH 8.8, 10% (w/v) acrylamide 0.1% (w/v) SDS, 0.05% (w/v) APS, 0.07% TEMED; stacking gel: 132 mM tris-HCl pH 6.8, 4% (w/v) acrylamide, 0.1% (w/v) SDS, 0.05% (w/v) APS, 0.15% (v/v) TEMED) were used to separate protein samples by gel electrophoresis. Separated proteins were transferred to PVDF membranes overnight at 4 o C. Blotted membranes were blocked with 5% Marvel semi-skimmed milk in TBST for 1 hour. Membranes were probed with primary antibodies (dilutions in parentheses): anti-LHCA4 (1:5000), RBCL (1:5000), UGPase (1:5000), PSBP1 (1:5000), D1/PSBA (1:5000), RPS1 (1:5000), RPS7 (1:5000), RPL2.1 (1:5000), RPL4 (1:5000), PetC (1:10 000) and NdhH (1:5000) (Agrisera- AS01 008, AS03 037 A, AS05 086, AS06 167, AS10 704, AS15 2875, AS15 2877, AS15 2876, AS15 3076, AS08 330 and AS16 4065); β-Glucuronidase (1:2000) (N-terminal (Sigma- G5420 ); GFP (1:5000) (Roche- 11814460001); Puromycin (1:10 000) (Merk- MABE343). All antibodies were diluted in TBST except for β-Glucuronidase (5% MILK-TBST), PetC (1% MILK-TBST) and NdhH (1% MILK-TBST)) and incubated for at least three hours (upto overnight). Membranes washed three times for 5 min in TBST and probed with appropriate secondary antibodies, anti-Rabbit-Hrp or anti-Mouse-Hrp (Sigma- A0545, A9917) diluted 1:5000 in TBST for one hour. Membranes were washed three times for 5 min in TBST then incubated with Pierce™ ECL Western Blotting Substrate (Thermo Scientific- 32106) for one minute. Membranes were exposed to X-ray film (FUJIFILM SUPER RX) in a HI-SPEED-X intensifying screen binder in a dark room. Films were developed with an Xograph Compact X4 Automated Processor and photographed on a light box with a Nikon D40 SLR camera. Immunoprecipitation PGR3-YFP fusion proteins were enriched from total protein extracts prepared from PGR3-YFP expressing col-0 and not4a plants with buffer containing proteasome and deubiquitinating enzyme inhibitors (Bortezomib and iodoacetamide) using GFP-Trap magnetic agarose beads (Chromotek- gtma-10) following the manufacturers procedure for washing and elution. Samples of the total protein extract and elution were analysed by western blotting with GFP (Roche- 11814460001) and ubiquitin (Abcam- ab18347) antibodies as detailed above. Chloroplast isolations Chloroplasts were isolated from short-day grown plants [84] . Two tubes containing 2 g of fresh rosette leaf per sample were mixed with 23 ml of chilled 1× isolation buffer each (0.6 M sorbitol, 0.1 M HEPES, 10 mM EDTA, 10 mM EGTA, 2 mM MgCl 2 , 20 mM NaHCO 3 and 1 mM DTT). Tissue was blended three times for 10 seconds with IKA T25 digital Ultra TURRAX at speed setting 3. Homogenate was poured into prewetted 38 µm pore polyester mesh and filtered again through double layer of prewetted 22 µm pore nylon cloth. Suspension was gently loaded onto two prepared falcon tubes containing equal volumes of 2× isolation buffer and Percoll TM (GE Healthcare- 17-0891-02). Samples were centrifuged in a swing bucket centrifuge at 1200 × g for 10 min with brakes off. Upper layers were and pellet washed with 8 ml 1× isolation buffer, inverting to mix. Samples were centrifuged again at 1000 × g for 5 min. Supernatants were removed using serological pipette and discarded. Pellets were resuspended in 5 ml 1× isolation buffer loaded gently onto a 50% percoll isolation buffer. Samples were centrifuged at 1200 × g for 10 min with brakes off. Upper layers removed with a serological pipette. Pellets were washed with 10 ml 1× isolation buffer, inverting to mix. Samples were centrifuged at 1000 × g for 5 and supernatant. Samples were centrifuged one final time at 1000 × g and remaining supernatant removed. Chloroplast pellets were frozen in liquid nitrogen. Proteins were solubilized in 2Xlaemmli buffer and quantified with the Biorad RC DC TM protein quantification assay. For chloroplast puromycin incorporation assays chloroplast enrichment was undertaken as above with the following adjustments: DTT excluded from isolation buffer. After the second percoll gradient chloroplast enriched pellets were washed once in resuspension buffer (1.6 M sorbitol, 0.1 M HEPES, 2.5 mM EDTA, 2.5 mM EGTA, 0.5 mM MgCl 2 , 20 mM NaHCO 3 ). Supernatants were removed and pellet resuspended in 2 ml of fresh resuspension buffer. 0.4 ml was taken for time-point 0 before adding 1.6 µl of 50 mM Puromycin dihydrochloride (Sigma- P8833), resuspensions were incubated in low light for 2 h, 0.4 ml was taken at each time-point and centrifuged at 12,000 × g for 1 min, supernatants removed and pellet snap frozen in liquid nitrogen. Protein extracts were prepared as above. Thylakoid composition analysis- Blue native and 2D gels Thylakoids were isolated from 5-week-old plants grown in 8-h light/ 16-h dark at photosynthetic photon flux density (PPFD) of 100 μmol m −2 s −1 , 50 % humidity, +23 °C, as described in ref. [85] . Protein concentration was determined using BioRad’s DC Protein assay according to the manufacturer’s protocol. Isolated thylakoids were diluted with ice-cold 25BTH20G [25 mM BisTris/HCl (pH 7.0), 20% (w/v) glycerol and 0.25 mg/ml Pefabloc, 10 mM NaF] buffer to a concentration of 10 mg protein/mL. An equal volume of detergent solution (β-dodecyl maltoside (DM) in BTH buffer) was added to a final concentration of 1% w/v. The membranes were solubilized 5 min on ice and the insolubilized material was removed by centrifugation at 18,000 × g at 4 °C for 20 min. The supernatant was supplemented with Serva Blue G buffer [100 mM BisTris/HCl (pH 7.0), 5 M ACA, 30%(w/v) sucrose and 50 mg/mL Serva Blue G] to introduce negative charge to the protein complexes. The Blue native (BN) gel (3.5–12.5% acrylamide) were prepared as described in Järvi et al., 2011 [37] . The protein complexes from the sample were separated by the BN gel and the individual subunits further resolved with 2D-SDS-PAGE (12% acrylamide, 6 M urea) as in Järvi et al., 2011 [37] . The proteins were visualized with SYPRO ® Ruby staining according to Invitrogen Molecular Probes™ instructions, or with silver staining [86] . Dual-PAM measurements Dual-PAM measurements were performed with Dual-PAM-100 (Heinz Walz GmbH) equipped with DUAL-E emitter and DUAL-DR detector units, using a red measuring beam for fluorescence and red actinic light. 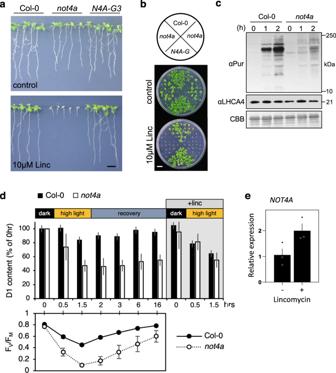Fig. 4: Plastid mRNA translation is compromised in thenot4amutant. a10-day-old WT,not4aandN4A-G3seedlings grown on vertical plates ±10 µM lincomycin. Bar = 1 cm.bsame as inabut on horizontal plates. Bar = 1 cm.cProtein synthesis rates in Col-0 andnot4achloroplasts, determined by anti-puromycin (α-Pur) western blot following a 2-h puromycin treatment time course. LHCA4 and CBB (Coomassie Brilliant blue) are shown as loading controls. Experiment was repeated at least three times with similar results.dThe amount of D1 protein (% of 0 h) and PSII efficiency (FV/FM) during a photoinhibitory treatment at 1000 μmol photons m−2s−1with and without lincomycin (linc) and during recovery without linc at 100 μmol photons m−2s−1. Total leaf protein extracts were separated on an SDS-PAGE, immunoblotted with a D1-specific antibody and quantified with LI-COR imaging. Averages from three biological replicates are presented with ±SEM error bars. Source data are included in the Source Data file.eQuantitative RT-PCR (qPCR) ofNOT4Ain 14-day-old Col-0 lines grown on media ±10 µM Lincomycin. Expression levels normalised toACTIN7and shown relative to untreated Col-0. Averages from three biological replicates are presented with ±SEM error bars. Simultaneously, the oxidation state of P700 was monitored by measuring the difference of the 875 nm and 830 nm transmittance signals. Prior to the measurements plants were dark-adapted for 30 min and F 0 , F M and P M were determined according to the Dual-PAM-100 protocol. For the light curve measurements the plants were subjected to illumination steps of 3 min at light intensities of 25–1000 μmol photons m −2 s −1 followed by a saturating flash (700 ms) to determine F M’ and P M’ . For the induction curve, dark-adapted plants were illuminated with 1000 μmol photons m −2 s −1 actinic light and a saturating flash was applied every 2 min. The quantum yield of PSII (Y(II)) was calculated [87] from the fluorescence data, while the P700 signal was used for the quantum yield of PSI (Y(I)) [88] . The relative rates of electron transfer through PSII and PSI, ETR(II) and ETR (I), respectively, were calculated as Y(II) × PPFD × 0.84 × 0.5 and Y(I) × PPFD × 0.84 × 0.5. Quantitative proteome analysis Col-0 and not4a plants were grown on ½ MS medium, supplemented with 0.8% sugar, for 30d under short-day conditions. Whole plants from three independent biological replicates was homogenized in Rensink extraction buffer (50 mM Tris/HCl pH 7.5, 100 mM NaCl, 0.5% (v/v) TritonX-100, 2 mM DTT and protease inhibitor cocktail (Sigma–Aldrich)). LC separation and HD-MSE data acquisition was performed as previously described by Helm et al., 2014 [40] . In short, 100 µg protein were digested in solution with RapiGestTM with 1 µg Trypsin (Promega) overnight. 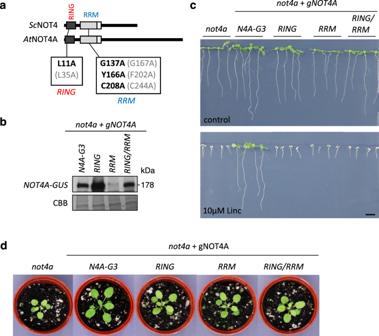Fig. 5: Functional domain analysis of NOT4A. aSchematic diagram showing position of point mutations in RING and RRM domains. Mutations in black are those introduced to theNOT4Agene, which correspond to equivalent conserved residues inScNOT4 (shown in grey), additionally highlighted in Supplementary Fig.1sequence alignments.banti-GUS western blot of steady state levels ofpNOT4A::NOT4A-GUS variants expressed innot4a. Blots were repeated at least three times with similar results.c10-day-oldnot4aandpNOT4A::NOT4A-GUS complementation lines grown on vertical plates ±10 µM lincomycin. Bar = 1 cm.dRepresentative rosette images of 3-week-oldnot4aandpNOT4A::NOT4A-GUS complementation lines under long day (LD) conditions. Bar = 1 cm. Peptide pellets were dissolved in 2% (v/v) ACN, 0.1% (v/v) FA, and subjected to LC on an ACQUITY UPLC System coupled to a Synapt G2-S mass spectrometer (Waters, Eschborn, Germany). For quantification, the sample was spiked with 10 fmol rabbit glycogen phosphorylase and the abundance of the three most intense peptide ions were used as s reference value for 10 fmol (Hi-3 method [89] . Data analysis and quantification was carried out by ProteinLynx Global Server (PLGS 3.0.1, Apex3D algorithm v. 2.128.5.0, 64 bit, Waters, Eschborn, Germany) with automated determination of chromatographic peak width as well as MS TOF resolution. Database query was as follows: Peptide and fragment tolerances were set to automatic, two fragment ion matches per peptide, five fragment ions for protein identification, and two peptides per protein were required for identification. Primary digest reagent was trypsin with one missed cleavage allowed. The false discovery rate (FDR) was set to 4% at the protein level. MSE data were searched against the modified A. thaliana database (TAIR10, ftp://ftp.arabidopsis.org ) containing common contaminants such as keratin ( ftp://ftp.thegpm.org/fasta/cRAP/crap.fasta ). All quantitative proteomics data were obtained with three independent biological replicates that were measured in three technical replicates each, giving rise to nine measurements per sample. Mapman was used to assign proteins to functional groups [90] . Statistical testing was based on a two-sided t -test [40] . Photoinhibition assays Detached leaves of mature plants grown under standard conditions for five weeks were floated on water or 2.3 mM lincomycin for 16 h in darkness after which they were illuminated under with high light of 1000 μmol photons m −2 s −1 for 1.5 h. Thereafter, the water samples were moved to standard growth conditions for recovery. PSII efficiency (F V /F M ) was measured after a 20 min dark-adaptation using FluorPen FP 110 (Photon Systems Instruments). The amount of D1 protein was measured by western blotting with protein samples collected at indicated timepoints. Total protein samples were isolated by homogenizing frozen leaf material in 100 mM Tris-HCl pH 8.0, 50 mM Na-EDTA, 0.25 mM NaCl, 0.75 (w/v) % SDS, 1 mM DTT followed by 10 min incubation at 68 °C. The extracts were clarified by centrifugation at 12,000 × g for 10 min. Protein concentration was determined using BioRad’s DC Protein assay according to the manufacturer’s protocol. Solubilized protein samples were separated by SDS-PAGE (12% acrylamide, 6 M urea) and immunoblotted with rabbit D1 DE-loop antibody [91] used as a 1:8000 dilution. LI-COR Goat anti-rabbit IRDye ® 800CW 2nd antibody was used for detection according to manufacturer’s instructions. Confocal microscopy Four-day-old pPGR3::PGR3-YFP expressing seedlings were imaged with a Nikon Ti microscope connected to an A1R confocal system equipped with a Plan Apochromat 60x/1.2 WI DIC H lens, with 514 nm and 637 nm laser lines, to image YFP and chlorophyll auto-fluorescence, respectively. Laser power, gain and pinhole settings used were identical between lines, YFP was imaged prior to chloroplast auto-fluorescence and settings compared to WT seedlings as a YFP negative control. At least four seedlings per genetic background were imaged. Yeast two-hybrid PGR3 and NOT4A coding sequences were cloned into Invitrogen pENTR™/D-TOPO™ (ThermoFisher- K240020) and sequenced before ligation into pGADCg and pGBKCg, respectively, (For primer sequences see, Supplementary Data 3 ). 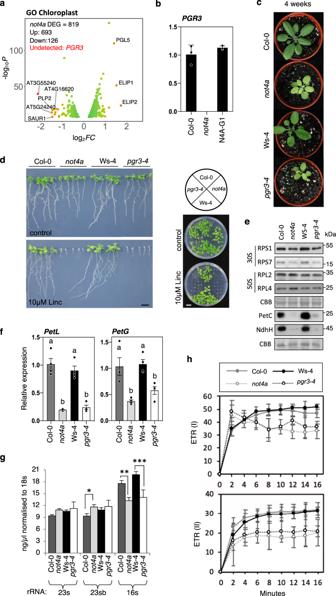Fig. 6: Thenot4amutant mimics thepgr3pentatricopeptide mutant. aVolcano plot of GO chloroplast-associated (GO:0009507) DEGs innot4avs WT. The top 8 DEGs are labelled (UP: ELIP2/AT4G14690, ELIP1/AT3G22840, PGL5/AT5G24420 and DOWN: AT3G55240, AT5G24240, SAUR1/AT4G34770, PLP2/AT2G26560, AT4G16620).bQuantitative PCR (qPCR) ofPGR3in Col-0,not4aandN4A-G3complementation line. Expression levels normalised toACTIN7and shown relative to Col-0 WT. Error bars = ±SEM.n= 3 biological replicates. Letters indicate one-way ANOVA; Tukey’s test (p< 0.01).cRepresentative rosette images of 4-week-old Col-0,not4a, Ws-4and pgr3-4lines grown under long day (LD) conditions. Bar = 1 cm.d10-day-old Col-0,not4a, Ws-4and pgr3-4seedlings grown on vertical and horizontal plates ±10 µM lincomycin. Bar = 1 cm.eWestern blot determination of 30 S ribosome subunits (RPS1 and RPS7), 50 S ribosome subunits (RPL2 and RPL4), PetC and NdhH in Col-0,not4a, Ws-4 andpgr3-4with coomassie blue (CBB) staining to show comparable protein loading. Blots were repeated at least three times with similar results.fqPCR ofPetL and PetGin 10-day old Col-0,not4a, Ws-4and pgr3-4seedlings. Expression levels normalised toACTIN7and shown relative to Col-0 WT. Data are average of three biological replicates. Letters indicate one-way ANOVA; Tukey’s test (p< 0.01). Error bars = ±SEM.gRelative amounts (ng/μl) of 50 S (23 s and 23 sb) and 30 S (16 s) plastid rRNAs in Col-0,not4a, Ws-4and pgr3-4seedlings. Values are quantified from Tapestation data shown in Supplementary Fig.5, following normalisation to cytosolic 18 s rRNA. Col-0 andnot4adata are same as in Fig.3e. Error bars = ±SEM.n= 3 biological replicates. *p= 0.0446, **p= 0.0037, ***p= 0.027, studentst-test, two-tailed.hETR(I) and ETR(II) during an induction curve measurement. Dark-adapted Col-0,not4a, Ws-4 andpgr3plants were illuminated with 1000 μmol photons m−2s−1actinic light and a saturating flash was applied every 2 min to determine FM’and PM’. The relative rates of electron transfer through PSI and PSII, ETR(I) and ETR (II), respectively, were calculated as in Fig.2. Each point represents the average ±SD (n= 3–4). 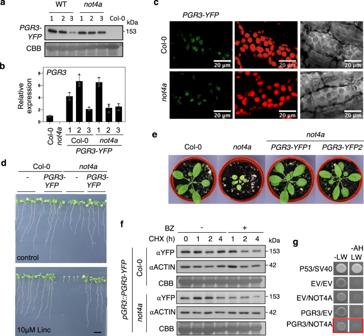Fig. 7: PGR3 can rescue the chloroplast-associated defects innot4a. aAnti-YFP western blot of steady state PGR3-YFP protein levels in three independent Col-0 andnot4alines expressingpPGR3::PGR3-YFP.bQuantitative PCR (qPCR) ofPGR3in Col-0,not4aand thePGR3-YFPlines froma. Expression levels normalised toACTIN7and shown relative to Col-0 WT.n= 3 biological replicates. Error bars = SEM.cConfocal images of hypocotyl cells in Col-0 andnot4alines expressingpPGR3::PGR3-YFP. Panels show PGR3-YFP in green (left), chloroplasts in red (middle) and bright field view (right). Experiment was replicated at least 3 times (see Supplementary Fig.7Dfor further repeats).d10-day-old Col-0,not4aand PGR3-YFP transgenic seedlings grown on vertical plates ±10 µM lincomycin. Bar = 1 cm.eRepresentative rosette images of 4-week-old Col-0,not4a and not4a PGR3-YFPlines grown under long day (LD) conditions. Bar = 1 cm.fCycloheximide (CHX) chase of PGR3-YFP and ACTIN in Col-0 andnot4a± bortezomib (BZ).gYeast two-hybrid assay between NOT4A and PGR3. EV empty vector. P53/SV40 positive control. Growth on -LW confirms successful transformation; growth on -AHLW denotes interaction. Western blots in 7a and 7f were repeated three times with similar results. Matchmaker (AH109) yeast was transformed with 1 µg pGADCg and pGBKCg vectors containing NOT4A, PGR3 or empty vectors as described, in 100 µl TB buffer (2:1 50% PEG 3350 MW, 1 M Lithium Acetate, 0.6% ß-mercaptoethanol). 37 °C for 45 min and then spread on agar plates containing yeast Nitrogen Base without Amino acids supplemented with synthetic amino acid Drop out (DO) -leu-trp agar (Formedium- CYN0401, DSCK172) and grown at 30 °C for 2–3 days before resuspending single colonies in 100 µl sterile water and transferring 20 µl to DO -leu-trp-his-ade and DO -leu-trp agar plates (Formedium- DSCK272, DSCK172). Plates were grown at 30 °C for 2–3 days before photographing with Nikon D40 SLR camera.